The class II PI 3-kinase, PI3KC2α, links platelet internal membrane structure to shear-dependent adhesive function PI3KC2α is a broadly expressed lipid kinase with critical functions during embryonic development but poorly defined roles in adult physiology. Here we utilize multiple mouse genetic models to uncover a role for PI3KC2α in regulating the internal membrane reserve structure of megakaryocytes (demarcation membrane system) and platelets (open canalicular system) that results in dysregulated platelet adhesion under haemodynamic shear stress. Structural alterations in the platelet internal membrane lead to enhanced membrane tether formation that is associated with accelerated, yet highly unstable, thrombus formation in vitro and in vivo. Notably, agonist-induced 3-phosphorylated phosphoinositide production and cellular activation are normal in PI3KC2α-deficient platelets. These findings demonstrate an important role for PI3KC2α in regulating shear-dependent platelet adhesion via regulation of membrane structure, rather than acute signalling. These studies provide a link between the open canalicular system and platelet adhesive function that has relevance to the primary haemostatic and prothrombotic function of platelets. Phosphoinositide 3-kinases (PI3Ks) are a family of enzymes that phosphorylate the 3′-OH position of the inositol ring of phosphatidylinositol (PI), generating 3-phosphorylated phosphoinositide (3-PPI) second messengers that regulate a broad range of signalling pathways (see ref. 1 for review). The 3-PPI lipids (PI(3)P, PI(3,4)P 2 and PI(3,4,5)P 3 ) bind PX, FYVE and PH domains of proteins to act as scaffolding complexes for intracellular signalling effectors, influencing the location and activity of a host of signalling complexes. The eight mammalian PI3K isoforms are separated into three subtypes based on their primary structure, lipid substrate specificity and mode of regulation. The four class I PI3Ks (p110 α, β, γ and δ) have well-characterized roles in a number of cellular functions including cell proliferation, survival, migration and intracellular protein trafficking (see ref. 2 for review), and much work has been aimed at targeting these enzymes for therapeutic use [3] . In this regard, we have previously shown that a series of isoform-selective inhibitors of the class I PI3K, p110β, impair platelet activation and prevent arterial thrombosis in vivo using rodent models and in human whole-blood thrombosis models [4] , [5] . These pharmacological studies were recently confirmed using genetically deficient mouse models [6] , [7] , indicating that the class I PI3K p110β has a critical role in platelet function during arterial thrombosis. In contrast to the class I PI3Ks, the roles of the class II PI3Ks (PI3KC2α, -C2β and -C2γ) have been less clearly defined, although recent studies have begun to shed light on their cellular functions. Both PI3KC2α and PI3KC2β (encoded by Pik3c2a and Pik3c2b , respectively) are widely expressed in mammalian cells, while PI3KC2γ expression is largely restricted to exocrine glands [8] . Pik3c2b −/− mice are healthy, fertile and appear phenotypically normal [9] , suggesting potential redundancy in class II PI3K function. Recently, Harris et al. [10] described mice harbouring a gene trapped hypomorphic allele of Pik3c2a that reduces PI3KC2α enzyme expression and activity by ~80%. Hypomorphic PI3KC2α mice displayed multiple phenotypes, including runting and impaired renal function [10] . Further, Yoshioka et al. [11] reported that complete deficiency of PI3KC2α results in an early and fully penetrant embryonic lethality due to defective vasculogenesis. Selective deletion of Pik3c2a in endothelial cells recapitulated this embryonic phenotype [11] . In combination with further work in isolated endothelial cells [12] , [13] , these studies strongly suggest that PI3KC2α is important in the setting of endothelial integrity and function during vascular development. The essential role for PI3KC2α in embryonic development may relate to the fundamental role of its lipid products, most likely PI(3)P and/or PI(3,4)P 2 , in regulating membrane dynamics, protein sorting and cell signalling. PI3KC2α is preferentially localized to clathrin-coated endocytic vesicles, other endosomes and the trans -Golgi network where it plays a major role in the regulation of vesicular trafficking [14] , [15] , [16] , and there is abundant evidence that the PI3K lipid product, PI(3)P, has the capacity to regulate the fusion, maturation and mobility of membranes [17] , [18] , [19] , [20] , [21] , [22] . Haematopoietic cells, particularly platelets and leukocytes, have evolved well-developed and often complex membrane systems that enable them to perform a variety of physiological functions linked to the maintenance of vascular integrity, host defence and tissue repair. Platelets and leukocytes are also notable for their extensive membrane reserves that provide a readily available source of lipid bilayer for rapid plasma membrane expansion [23] , [24] . These membrane reservoirs are present as either invaginations of the plasma membrane (for example, the open canalicular system (OCS) in platelets) or as external folds (for example, macrophage microvilli). In haematopoietic cells, mobilization of membrane reserves is important for the development of membrane tethers, filopodia and lamellae extensions at the leading edge of migrating cells, phagocytosis and the prevention of cell lysis during osmotic stress [25] , [26] . The internal membrane reserves of the platelet, known as the surface-connected OCS, consists of a network of membrane-bound cisternae and tubules [27] . It is a dominant ultrastructural feature of the cell and plays a key role in the morphological changes critical for platelet function (for review, see ref. 24 ). Despite this important function, our understanding of the molecular mechanisms regulating platelet internal membranes remains rudimentary. We report here a novel function for PI3KC2α in regulating the structure of the internal membrane reserves of platelets and megakaryocytes. We generate a series of new genetic mouse models in which PI3KC2α is markedly reduced and observe that altered structure of the demarcation membrane system (DMS) of PI3KC2α-deficient megakaryocytes does not impact on quantitative platelet production, but that altered structure of the platelet OCS leads to dysregulated platelet adhesion and the consequent formation of large, unstable platelet thrombi. These studies define an unexpected role for PI3KC2α in regulating the structure of the platelet internal membranes, and provide the first evidence linking the OCS to the haemostatic and prothrombotic function of platelets. PI3KC2α is important for mouse platelet function in vivo We determined the class II PI3K protein expression profile in platelets from both mice and humans. We observed expression of PI3KC2α and PI3KC2β, but not PI3KC2γ, in platelets from both species ( Fig. 1a ), consistent with previous findings that PI3KC2α and PI3KC2β are more broadly expressed than PI3KC2γ [28] , [29] Based on our expression analysis ( Fig. 1a ) and a previous biochemical study in isolated cells [30] , PI3KC2β appeared the dominant class II PI3K isoform in platelets, where it has been proposed to produce PI(3,4)P 2 in response to platelet activation and consequent integrin α IIb β 3 ligation [30] . However, detailed analysis of 3-PPIs in unstimulated and agonist-activated platelets from Pik3c2b −/− mice revealed no significant differences in the levels of PI(3)P, PI(3,4)P 2 or PI(3,4,5)P 3 relative to littermate Pik3c2b +/+ controls ( Fig. 1b ). Furthermore, analysis of a broad range of platelet functional responses, including agonist-induced platelet aggregation, shape change, integrin α IIb β 3 activation and release of either alpha or dense granules, revealed no significant differences in platelets isolated from littermate Pik3c2b −/− and Pik3c2b +/+ mice ( Supplementary Fig. 1a–e ). The lack of effect of PI3KC2β deficiency on the rate and extent of platelet 3-PPI production and cell function was observed in response to activation via either a G-protein-coupled receptor (activation of protease-activated receptor 4 with thrombin) or an immune-type receptor (activation of GPVI with collagen-related peptide (CRP)). In keeping with normal platelet function, Pik3c2b −/− mice had a normal haemostatic response following tail transection ( Supplementary Fig. 1f ) and a normal thrombotic response following electrolytic injury of the carotid artery ( Supplementary Fig. 1g ). Together, these studies indicate that PI3KC2β is not absolutely required for 3-PPI production in platelets or for activation pathways important for the haemostatic and prothrombotic function of mouse platelets in vivo . 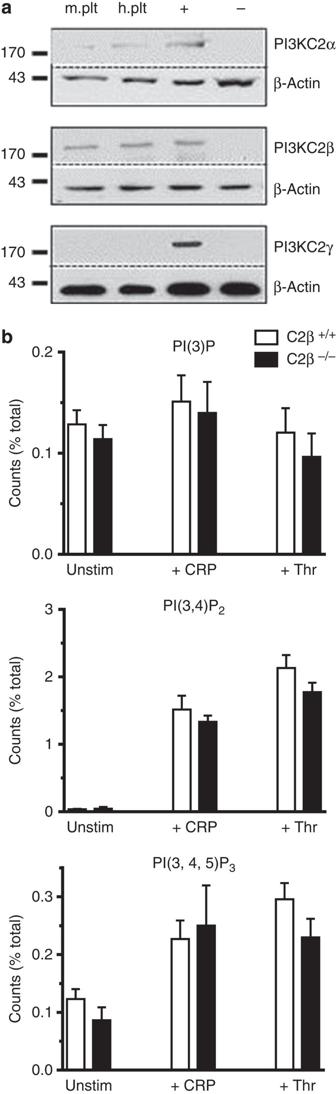Figure 1: Expression and functional analysis of PI3KC2β in mouse platelets. (a) Immunoblots for all three class II PI3Ks, PI3KC2α, PI3KC2β and PI3KC2γ, on lysates of platelets isolated from mice (m. plt) and humans (h. plt). Note that the number of platelets used for lysates in the PI3KC2α and PI3KC2γ blots is 10 times that of the PI3KC2β blot. Positive controls (+) are mouse brain for PI3KC2α and PI3KC2γ, and liver for PI3KC2β. Negative controls (−) arePik3c2a−/−embryos,Pik3c2b−/−liver and NIH3T3 for PI3KC2γ. Immunoblots for β-actin and the respective PI3Ks were performed on the same membranes. Data are representative of ≥4 independent experiments. (b) Quantification of high-performance liquid chromatography-based analysis of 3-PPI generation in platelets isolated from WT (C2β+/+) andPik3c2b−/−(C2β−/−) mice. Platelets were treated with vehicle (unstimulated, unstim), 10 μg ml−1collagen-related peptide (+CRP) or 1 U ml−1thrombin (+Thr) for 5 min. Data are expressed as a percentage of the total phosphorylated lipid content in individual samples and are mean±s.e.m. ofn=4–9 independent experiments (mice). No significant differences were detected by genotype at any point (unpaired, two-tailed, Student’st-test). Note that similar 3-PPI analyses performed at 0.25, 0.5, 1 and 2 min post stimulation also failed to reveal differences by genotype and are not shown for simplicity of the figure. Figure 1: Expression and functional analysis of PI3KC2β in mouse platelets. ( a ) Immunoblots for all three class II PI3Ks, PI3KC2α, PI3KC2β and PI3KC2γ, on lysates of platelets isolated from mice (m. plt) and humans (h. plt). Note that the number of platelets used for lysates in the PI3KC2α and PI3KC2γ blots is 10 times that of the PI3KC2β blot. Positive controls (+) are mouse brain for PI3KC2α and PI3KC2γ, and liver for PI3KC2β. Negative controls (−) are Pik3c2a −/− embryos, Pik3c2b −/− liver and NIH3T3 for PI3KC2γ. Immunoblots for β-actin and the respective PI3Ks were performed on the same membranes. Data are representative of ≥4 independent experiments. ( b ) Quantification of high-performance liquid chromatography-based analysis of 3-PPI generation in platelets isolated from WT (C2β +/+ ) and Pik3c2b −/− (C2β −/− ) mice. Platelets were treated with vehicle (unstimulated, unstim), 10 μg ml −1 collagen-related peptide (+CRP) or 1 U ml −1 thrombin (+Thr) for 5 min. Data are expressed as a percentage of the total phosphorylated lipid content in individual samples and are mean±s.e.m. of n =4–9 independent experiments (mice). No significant differences were detected by genotype at any point (unpaired, two-tailed, Student’s t -test). Note that similar 3-PPI analyses performed at 0.25, 0.5, 1 and 2 min post stimulation also failed to reveal differences by genotype and are not shown for simplicity of the figure. Full size image The role of PI3KC2α in platelets has not been examined previously. To investigate the possibility of redundancy in class II PI3K function in platelets, we generated mice with a single or combined PI3KC2α/β deficiency. Two PI3KC2α mutant mouse lines were generated, carrying independent gene trapped alleles of Pik3c2a —one 5′ ( Pik3c2a gt1 ) and one 3′ ( Pik3c2a gt2 ) of the region encoding the catalytic domain, and predicted to yield a truncated fusion protein of the first 837 or 1,029 amino acids of PI3KC2α linked to β-galactosidase, respectively ( Fig. 2a,b ). Similar to a recent report [11] , we found that 100% of Pik3c2a gt1/gt1 and Pik3c2a gt2/gt2 mice died in utero , with growth retardation from 6.5 days post coitum (dpc) and no development beyond 8.5 dpc ( Fig. 2c and Table 1 ). Both Pik3c2a +/gt1 and Pik3c2a +/gt1 ; Pik3c2b −/− mice were born at expected numbers, showed no gross abnormalities and had platelets that were normal in number and size ( Supplementary Fig. 2 ). While Pik3c2a +/gt1 ; Pik3c2b −/− mice exhibited no overt functional platelet defects in a range of in vitro assays ( Supplementary Fig. 3 ), they exhibited a prolonged bleeding time in a sensitized tail bleeding assay using hirudin ( Fig. 3a ). Anticoagulation with hirudin alone (5 mg kg −1 ) has no impact on tail bleeding time but increases the sensitivity of the bleeding time to primary platelet haemostatic defects. Strikingly, loss of a single allele of Pik3c2a ( Pik3c2a +/gt1 ) also resulted in a prolongation in tail bleeding under these conditions ( Fig. 3a ). In contrast, Pik3c2b −/− mice were unaffected ( Fig. 3a ). The prolonged bleeding was observed with both PI3KC2α-deficient mouse lines, and the increase in bleeding time was similar in magnitude to that observed in mice pretreated with the antiplatelet drug, aspirin ( Fig. 3a ). 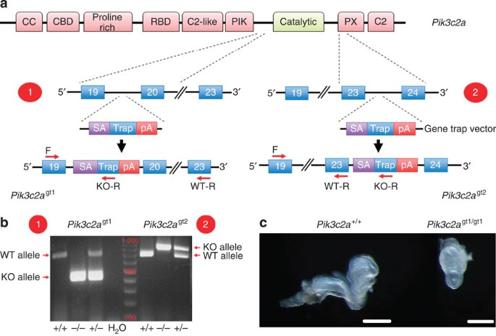Figure 2: Generation ofPik3c2a−/−mice. (a) Schematic of the gene trap mutation and genotyping strategy for disruption ofPik3c2ain mice. Two distinct truncations ofPik3c2awere generated—one 5′ (1:Pik3c2agt1) and one 3′ (2:Pik3c2agt2) of the region encoding the catalytic domain (green box). Insertion of a gene trap vector encoding a splice acceptor (SA) β-galactosidase (trap) and a polyA stop site (pA) into thePik3c2alocus occurred either between exons 19 and 20 (Pik3c2agt1) or exons 23 and 24 (Pik3c2agt2), and is predicted to yield a truncated fusion protein of the first 837 or 1,029 amino acids of PI3KC2α linked to β-galactosidase, respectively. Red arrows indicate positions of the genotyping primers (F=common forward; KO-R=knockout reverse; WT-R=wildtype reverse), which were common to both mutations. (b) Representative genotypic analysis of embryos via RT–PCR using the strategy depicted, with the predicted single band of either 460 or 830 bp inPik3c2agt1/gt1andPik3c2agt2/gt2embryos respectively, a single band of 750 bp inPik3c2a+/+embryos, and both bands inPik3c2a+/gt1andPik3c2a+/gt2embryos. (c) Representative whole-mount pictures of littermatePik3c2a+/+orPik3c2agt1/gt1embryos fromPik3c2a+/gt1intercrosses at 8.5 days post coitum, showing markedly delayed development inPik3c2agt1/gt1embryos. Scale bars=1 mm. Figure 2: Generation of Pik3c2a −/− mice. ( a ) Schematic of the gene trap mutation and genotyping strategy for disruption of Pik3c2a in mice. Two distinct truncations of Pik3c2a were generated—one 5′ (1: Pik3c2a gt1 ) and one 3′ (2: Pik3c2a gt2 ) of the region encoding the catalytic domain (green box). Insertion of a gene trap vector encoding a splice acceptor (SA) β-galactosidase (trap) and a polyA stop site (pA) into the Pik3c2a locus occurred either between exons 19 and 20 ( Pik3c2a gt1 ) or exons 23 and 24 ( Pik3c2a gt2 ), and is predicted to yield a truncated fusion protein of the first 837 or 1,029 amino acids of PI3KC2α linked to β-galactosidase, respectively. Red arrows indicate positions of the genotyping primers (F=common forward; KO-R=knockout reverse; WT-R=wildtype reverse), which were common to both mutations. ( b ) Representative genotypic analysis of embryos via RT–PCR using the strategy depicted, with the predicted single band of either 460 or 830 bp in Pik3c2a gt1/gt1 and Pik3c2a gt2/gt2 embryos respectively, a single band of 750 bp in Pik3c2a +/+ embryos, and both bands in Pik3c2a +/gt1 and Pik3c2a +/gt2 embryos. ( c ) Representative whole-mount pictures of littermate Pik3c2a +/+ or Pik3c2a gt1/gt1 embryos from Pik3c2a +/gt1 intercrosses at 8.5 days post coitum, showing markedly delayed development in Pik3c2a gt1/gt1 embryos. Scale bars=1 mm. Full size image Table 1 Genotype analysis of embryos generated from Pik3c2a +/− intercrosses. 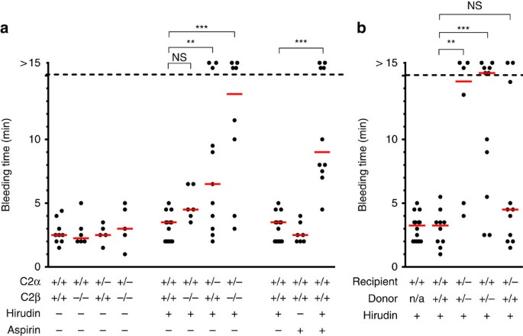Figure 3: PI3KC2α is important for mouse platelet functionin vivo. (a) Tail bleeding times, determined using the template method, in an allelic series of PI3KC2-deficient mice in the absence and presence of the anticoagulant, hirudin (5 mg kg−1), and in WT mice treated with hirudin (5 mg kg−1), aspirin (200 mg kg−1) or both drugs. Note that bleeding is prolonged only in hirudin-anticoagulated mice that were at a minimum heterozygous forPik3c2a, and that the extent of this bleeding was similar to hirudin-anticoagulated WT mice treated with a therapeutic dose of the standard antiplatelet agent, aspirin33,63. (b) Tail bleeding times in anticoagulated chimaeric mice 8 weeks after bone marrow transplantation. Recipient mice reconstituted withPik3c2a+/gt1donor marrow (+/−) had significantly prolonged tail bleeding times versus those reconstituted with WT (+/+) marrow. Chimaerism was determined via CD45 isotype expression as >90% in all cases. Data points represent time to cessation of bleeding in an individual mouse following a defined incision in the tail. Experiments were terminated after 15 min, with mice still bleeding at this time shown above the dotted line. Red bars are medians. Significance was determined after plotting the same data as Kaplan–Meier survival curves and analysing by log-rank test with a Bonferroni correction for multiple comparisons versus the indicated control group (**P<0.01; ***P<0.001; NS, not significant.) Full size table Figure 3: PI3KC2α is important for mouse platelet function in vivo. ( a ) Tail bleeding times, determined using the template method, in an allelic series of PI3KC2-deficient mice in the absence and presence of the anticoagulant, hirudin (5 mg kg −1 ), and in WT mice treated with hirudin (5 mg kg −1 ), aspirin (200 mg kg −1 ) or both drugs. Note that bleeding is prolonged only in hirudin-anticoagulated mice that were at a minimum heterozygous for Pik3c2a , and that the extent of this bleeding was similar to hirudin-anticoagulated WT mice treated with a therapeutic dose of the standard antiplatelet agent, aspirin [33] , [63] . ( b ) Tail bleeding times in anticoagulated chimaeric mice 8 weeks after bone marrow transplantation. Recipient mice reconstituted with Pik3c2a +/gt1 donor marrow (+/−) had significantly prolonged tail bleeding times versus those reconstituted with WT (+/+) marrow. Chimaerism was determined via CD45 isotype expression as >90% in all cases. Data points represent time to cessation of bleeding in an individual mouse following a defined incision in the tail. Experiments were terminated after 15 min, with mice still bleeding at this time shown above the dotted line. Red bars are medians. Significance was determined after plotting the same data as Kaplan–Meier survival curves and analysing by log-rank test with a Bonferroni correction for multiple comparisons versus the indicated control group (** P <0.01; *** P <0.001; NS, not significant.) Full size image Since PI3KC2α was recently demonstrated to play an important role in regulating endothelial cell barrier function and vasculogenesis [11] , we examined tail bleeding times on chimaeric mice generated via bone marrow transplantation in order to confirm that the prolonged bleeding in Pik3c2a +/gt1 mice was intrinsic to haematopoietic cells. There was a nonsignificant trend towards increased bleeding in Pik3c2a +/gt1 -recipient mice transplanted with Pik3c2a +/+ donor marrow ( Fig. 3b ). In contrast, impaired haemostasis was observed in Pik3c2a +/+ recipients transplanted with haematopoietic cells taken from Pik3c2a +/gt1 mice that was similar in magnitude to that observed in the control transplant of Pik3c2a +/gt1 haematopoietic cells into Pik3c2a +/gt1 recipients ( Fig. 3b ). While we cannot exclude the possibility that vascular dysfunction contributes to the prolonged tail bleeding in Pik3c2a +/gt1 mice, these findings strongly suggest a platelet defect as the most significant cause of the increased bleeding in these animals. PI3KC2α deficiency exacerbates bleeding and impairs thrombosis To circumvent the embryonic lethality of mice with a global deficiency in PI3KC2α, we adopted an RNAi-based approach to inducibly deplete PI3KC2α expression in vivo ( Fig. 4a ). We used a recently developed targeting strategy to generate transgenic mice where a tetracycline (tet)-regulated promoter controls co-expression of green fluorescent protein (GFP) and an short hairpin RNA (shRNA) targeting mouse PI3KC2α (TRE-GFP-shPI3KC2α mice). To induce shRNA expression in these mice, we crossed them to a transgenic mouse strain expressing the reverse tet transactivator protein rtTA (tet-on) under control of the cytomegalovirus (CMV) promoter (CMV-rtTA mice), which we have previously shown drives effective and inducible protein reduction in platelets of adult mice [31] . As anticipated, doxycycline treatment of CMV-rtTA;TRE-GFP-shPI3KC2α bitransgenic mice (hereafter referred to as shPI3KC2α) resulted in a time-dependent increase in the percentage of GFP+ platelets, indicating expression of shPI3KC2α, which plateaued beyond 9 days at ≥95% ( Supplementary Fig. 4 ). This resulted in a concomitant reduction in PI3KC2α protein levels in circulating platelets isolated from these mice ( Fig. 4b ). Persistent knockdown of PI3KC2α by continuous doxycycline administration (up to 2 months) had no detrimental effect on mouse viability, caused no biochemical changes suggestive of major organ injury and blood cell counts remained in the normal range. However, direct comparison of in vivo haemostasis between shPI3KC2α mice and their littermate wild-type (WT) or monotransgenic controls revealed a significant prolongation in tail bleeding time in all 10 shPI3KC2α mice examined ( Fig. 4c ). In contrast, doxycycline-dependent induction of a control shRNA had no impact on bleeding time ( Fig. 4c ). Comparing the tail bleeding times of four distinct mouse lines with varying levels of PI3KC2α deficiency ( Pik3c2a +/gt1 , Pik3c2a +/gt2 , a previously described hypomorphic Pik3c2a allele [10] and the shPI3KC2α mice) revealed a strong correlation between PI3KC2α expression and in vivo platelet function ( Fig. 4d ). 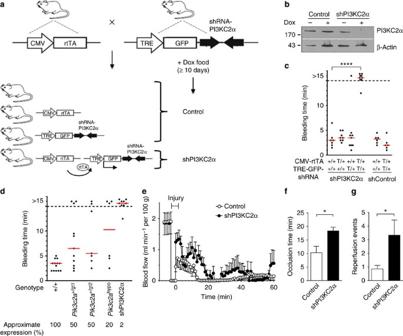Figure 4: PI3KC2α deficiency exacerbates bleeding and impairs thrombosis. (a) Schematic of the experimental strategy used to inducibly inhibit PI3KC2α expressionin vivo. CMV-rtTA;TRE-GFP-shPI3KC2α bi-transgenic mice (shPI3KC2α) and littermate controls (control=pooled WT and monotransgenic) were fed doxycycline-containing food (600 mg kg−1) for ≥10 days before experimentation. (b) Western blot showing expression of PI3KC2α and β-actin in platelets derived from shPI3KC2α and littermate controls. Immunoblots for PI3KC2α and β-actin were performed on the same membranes. Data are representative of three independent experiments. (c) Tail bleeding times in anticoagulated (hirudin; 5 mg kg−1) shPI3KC2α and littermate control mice, as well as those expressing a control shRNA targeting Renilla luciferase (shControl). All mice were exposed to doxycycline-containing food for ≥10 days. (d) Tail bleeding times in four distinct PI3KC2α-deficient mouse lines: WT (+/+), the two gene trap-mediated PI3KC2α+/−lines generated in this study (Pik3c2a+/gt1andPik3c2a+/gt2), a previously described hypomorphic PI3KC2α allele (Pik3c2ahypo)10and shPI3KC2α mice. Note that some data provided here is reproduced fromFigs 3aand4c. Inc,d, data points represent time to cessation of bleeding in an individual mouse following a defined incision in the tail. Experiments were terminated after 15 min, with mice still bleeding at this time shown above the dotted line. Red bars are medians. Significance was determined after plotting the same data as Kaplan–Meier survival curves and analysing by log-rank test with a Bonferroni correction for multiple comparisons versus the control group (****P<0.0001). (e–g)In vivothrombosis in shPI3KC2α (closed symbols) and littermate control mice (pooled WT and monotransgenic littermates; open symbols). Electrolytic injury of carotid arteries was induced under stasis by a current of 18 mA for 2 min (injury). Shown are (e) blood flow rates from 5 min before to 60 min after injury, (f) mean time to first occlusion (zero blood flow recorded for >2 min), and (g) average number of reperfusion events during the 60-min observation period. Data are mean±s.e.m.;n=6–7. *P<0.05. Figure 4: PI3KC2α deficiency exacerbates bleeding and impairs thrombosis. ( a ) Schematic of the experimental strategy used to inducibly inhibit PI3KC2α expression in vivo . CMV-rtTA;TRE-GFP-shPI3KC2α bi-transgenic mice (shPI3KC2α) and littermate controls (control=pooled WT and monotransgenic) were fed doxycycline-containing food (600 mg kg −1 ) for ≥10 days before experimentation. ( b ) Western blot showing expression of PI3KC2α and β-actin in platelets derived from shPI3KC2α and littermate controls. Immunoblots for PI3KC2α and β-actin were performed on the same membranes. Data are representative of three independent experiments. ( c ) Tail bleeding times in anticoagulated (hirudin; 5 mg kg −1 ) shPI3KC2α and littermate control mice, as well as those expressing a control shRNA targeting Renilla luciferase (shControl). All mice were exposed to doxycycline-containing food for ≥10 days. ( d ) Tail bleeding times in four distinct PI3KC2α-deficient mouse lines: WT (+/+), the two gene trap-mediated PI3KC2α +/− lines generated in this study ( Pik3c2a +/gt1 and Pik3c2a +/gt2 ), a previously described hypomorphic PI3KC2α allele ( Pik3c2a hypo ) [10] and shPI3KC2α mice. Note that some data provided here is reproduced from Figs 3a and 4c . In c , d , data points represent time to cessation of bleeding in an individual mouse following a defined incision in the tail. Experiments were terminated after 15 min, with mice still bleeding at this time shown above the dotted line. Red bars are medians. Significance was determined after plotting the same data as Kaplan–Meier survival curves and analysing by log-rank test with a Bonferroni correction for multiple comparisons versus the control group (**** P <0.0001). ( e – g ) In vivo thrombosis in shPI3KC2α (closed symbols) and littermate control mice (pooled WT and monotransgenic littermates; open symbols). Electrolytic injury of carotid arteries was induced under stasis by a current of 18 mA for 2 min (injury). Shown are ( e ) blood flow rates from 5 min before to 60 min after injury, ( f ) mean time to first occlusion (zero blood flow recorded for >2 min), and ( g ) average number of reperfusion events during the 60-min observation period. Data are mean±s.e.m. ; n =6–7. * P <0.05. Full size image To investigate whether PI3KC2α deficiency also impacted on the prothrombotic function of platelets, we examined arterial thrombus formation in vivo following electrolytic injury of the carotid artery. When compared with littermate controls, the mean time to vessel occlusion by arterial thrombi was significantly greater in shPI3KC2α mice ( Fig. 4e,f ). Furthermore, the thrombi formed in shPI3KC2α mice were unstable, leading to a significant increase in spontaneous thromboembolism and intermittent vascular reperfusion ( Fig. 4e,g ). PI3KC2α deficiency alters platelet internal membrane structure To gain insight into the mechanisms leading to the impaired in vivo platelet function in PI3KC2α-deficient mice, we examined changes in 3-PPI levels, cell morphology and functional responses in isolated platelets. Detailed analysis of PI(3)P, PI(3,4)P 2 and PI(3,4,5)P 3 revealed no significant differences in the levels of these lipids in unstimulated or agonist-stimulated platelets isolated from either Pik3c2a +/gt1 or shPI3KC2α mice compared with their respective littermate controls ( Fig. 5a ). Moreover, a broad range of platelet functional responses, including platelet aggregation, integrin α IIb β 3 activation and release of either alpha or dense granules, were all normal in Pik3c2a +/gt1 and shPI3KC2α platelets in response to multiple platelet agonists ( Supplementary Figs 5 and 6 ). However, ultrastructure analysis of PI3KC2α-deficient platelets by transmission electron microscopy revealed enlarged ‘vacuolar’ structures ( Fig. 5b,c ) that were identified as the OCS by positive ruthenium red staining of surface-connected membranes ( Fig. 5d ). The OCS represents invaginations of the platelet plasma membrane and constitutes up to 50% of the cell’s total plasma membrane [32] . Both Pik3c2a +/gt1 and shPI3KC2α platelets displayed regions of dilated OCS, with a cross-sectional surface area that was 30–40% larger than in platelets from their respective littermates ( Fig. 5c ). This altered OCS structure occurred without any gross changes in the number or structure of other organelles or the actin cytoskeleton ( Supplementary Fig. 7 ), and suggests a specific role for PI3KC2α in regulating the structure of the internal membrane reserves of platelets that may underlie the impaired primary haemostatic and prothrombotic function of these cells. 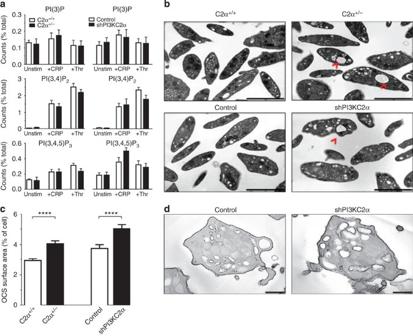Figure 5: PI3KC2α deficiency alters the platelet internal membrane structure. (a) Quantification of high-performance liquid chromatography-based analysis of 3-PPI generation in platelets isolated from littermate WT (C2α+/+) andPik3c2a+/gt1(C2α+/−) mice, and littermate CMV-rtTA;TRE-GFP-shPI3KC2α (shPI3KC2α) and control mice (control=pooled WT and monotransgenic). Platelets were treated with vehicle (unstimulated, unstim), 10 μg ml−1collagen-related peptide (+CRP) or 1 U ml−1thrombin (+Thr) for 5 min. Data are expressed as a percentage of the total phosphorylated lipid content of individual samples and are mean±s.e.m. ofn=3–7 independent experiments (mice). No significant differences were observed by genotype at any point (unpaired, two-tailed, Student’st-test). Similar analyses at 0.25, 0.5, 1 and 2 min post stimulation also failed to reveal differences by genotype and are not shown for simplicity of the figure. (b) Representative TEM images (n=4) of platelets isolated from littermate C2α+/+and C2α+/−mice, and littermate shPI3KC2α and control mice. Note the dilated OCS (red arrow heads) in platelets from both PI3KC2α-deficient mouse lines. (c) Quantification of OCS surface area. Data are expressed as a percentage of the total cell area and presented as mean±s.e.m. ofn=311–417 cells fromn=4 mice per genotype. ****P<0.0001 (unpaired, two-tailed, Student’st-test). (d) Representative TEM images (n=3) of platelets isolated from littermate shPI3KC2α and control mice pre-stained with ruthenium red. Note staining of the internal membrane structures in both cases, indicating surface connection. Scale bars, 2 μm (b) and 500 nm (d). Figure 5: PI3KC2α deficiency alters the platelet internal membrane structure. ( a ) Quantification of high-performance liquid chromatography-based analysis of 3-PPI generation in platelets isolated from littermate WT (C2α +/+ ) and Pik3c2a +/gt1 (C2α +/− ) mice, and littermate CMV-rtTA;TRE-GFP-shPI3KC2α (shPI3KC2α) and control mice (control=pooled WT and monotransgenic). Platelets were treated with vehicle (unstimulated, unstim), 10 μg ml −1 collagen-related peptide (+CRP) or 1 U ml −1 thrombin (+Thr) for 5 min. Data are expressed as a percentage of the total phosphorylated lipid content of individual samples and are mean±s.e.m. of n =3–7 independent experiments (mice). No significant differences were observed by genotype at any point (unpaired, two-tailed, Student’s t -test). Similar analyses at 0.25, 0.5, 1 and 2 min post stimulation also failed to reveal differences by genotype and are not shown for simplicity of the figure. ( b ) Representative TEM images ( n =4) of platelets isolated from littermate C2α +/+ and C2α +/− mice, and littermate shPI3KC2α and control mice. Note the dilated OCS (red arrow heads) in platelets from both PI3KC2α-deficient mouse lines. ( c ) Quantification of OCS surface area. Data are expressed as a percentage of the total cell area and presented as mean±s.e.m. of n =311–417 cells from n =4 mice per genotype. **** P <0.0001 (unpaired, two-tailed, Student’s t -test). ( d ) Representative TEM images ( n =3) of platelets isolated from littermate shPI3KC2α and control mice pre-stained with ruthenium red. Note staining of the internal membrane structures in both cases, indicating surface connection. Scale bars, 2 μm ( b ) and 500 nm ( d ). Full size image The structural defect coupled with the lack of signalling-dependent effects in PI3KC2α-deficient platelets suggested that the internal membrane changes in these cells may be inherited from the megakaryocyte. In support of this hypothesis, transmission electron microscopy analysis of in situ bone marrow megakaryocytes revealed a similar ultrastructural change in the internal membrane system of PI3KC2α-deficient megakaryocytes ( Fig. 6a ). Furthermore, expression of PI3KC2α was markedly greater in megakaryocytes relative to platelets ( Fig. 6b ). Indeed, PI3KC2α was difficult to detect by western blot in mouse platelets ( Fig. 6b ). Yet despite a dilated DMS in 68% of megakaryocytes in shPI3KC2α mice, no impact on megakaryocyte development or platelet production was observed: shPI3KC2α mice had normal megakaryocyte numbers in the bone marrow and spleen ( Fig. 6b ), and bone marrow-derived megakaryocytes exhibited normal ploidy ( Fig. 6c ) and proplatelet-producing capacity in culture ( Fig. 6d ). Furthermore, in vivo platelet half-life ( Fig. 6e ) and production following immune-mediated depletion ( Fig. 6f ) revealed no difference between shPI3KC2α and littermate WT mice. Since the altered DMS of PI3KC2α-deficient megakaryocytes did not impact on platelet production, we focussed on determining how the altered OCS of PI3KC2α-deficient platelets impacted platelet function. 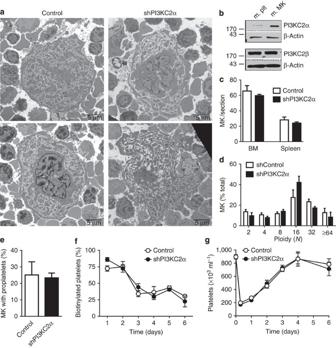Figure 6: PI3KC2α deficiency alters the megakaryocyte internal membrane structure. (a) Representative TEM images (n=6) ofin situbone marrow megakaryocytes (MKs) from littermate CMV-rtTA;TRE-GFP-shPI3KC2α (shPI3KC2α) and control mice (control=pooled WT and monotransgenic). Note the dilated DMS in MKs from PI3KC2α-deficient mice. Scale bars, 5 μm. (b) Immunoblots for PI3KC2α and PI3KC2β in mouse platelet and megakaryocyte samples matched for β-actin expression, showing limited comparative expression of PI3KC2α in platelets. (c) Quantification of MK numbers in sections of bone marrow (BM) and spleen. (d) Ploidy analysis of BM MKs. (e) Analysis of proplatelet production by BM-derived MKs after 5 days in culture. (f)In vivoplatelet lifespan and (g) platelet production following immune-mediated depletion in littermate CMV-rtTA;TRE-GFP-shPI3KC2α (shPI3KC2α) and control mice (control=pooled WT and monotransgenic). All data are mean±s.e.m. ofn=3–8 mice per genotype. No significant differences were observed by genotype at any point (unpaired, two-tailed, Student’st-test). Figure 6: PI3KC2α deficiency alters the megakaryocyte internal membrane structure. ( a ) Representative TEM images ( n =6) of in situ bone marrow megakaryocytes (MKs) from littermate CMV-rtTA;TRE-GFP-shPI3KC2α (shPI3KC2α) and control mice (control=pooled WT and monotransgenic). Note the dilated DMS in MKs from PI3KC2α-deficient mice. Scale bars, 5 μm. ( b ) Immunoblots for PI3KC2α and PI3KC2β in mouse platelet and megakaryocyte samples matched for β-actin expression, showing limited comparative expression of PI3KC2α in platelets. ( c ) Quantification of MK numbers in sections of bone marrow (BM) and spleen. ( d ) Ploidy analysis of BM MKs. ( e ) Analysis of proplatelet production by BM-derived MKs after 5 days in culture. ( f ) In vivo platelet lifespan and ( g ) platelet production following immune-mediated depletion in littermate CMV-rtTA;TRE-GFP-shPI3KC2α (shPI3KC2α) and control mice (control=pooled WT and monotransgenic). All data are mean±s.e.m. of n =3–8 mice per genotype. No significant differences were observed by genotype at any point (unpaired, two-tailed, Student’s t -test). Full size image PI3KC2α deficiency causes unstable platelet thrombi We examined platelet thrombus dynamics in PI3KC2α-deficient mice ex vivo by perfusing anticoagulated whole blood over an immobilized type I fibrillar collagen substrate [33] , [34] . Although the in vivo platelet function impairment was greater in shPI3KC2α mice, we focussed on Pik3c2a +/gt1 mice in these ex vivo whole-blood studies because we observed a genotype-independent increase in platelet adhesion in mice treated with doxycycline that artificially increased baseline values in these assays. Strikingly, in whole blood from Pik3c2a +/gt1 mice, the rate and extent of platelet thrombus formation was more rapid than in littermate Pik3c2a +/+ controls ( Fig. 7a ). Notably, the extent of the initial platelet–collagen interaction was indistinguishable between Pik3c2a +/+ and Pik3c2a +/gt1 mice (measured as thrombus adhesion area by confocal microscopy; Fig. 7b ); however, the size of individual platelet thrombi was greater in Pik3c2a +/gt1 mice relative to littermate controls (measured as thrombus height and volume by confocal microscopy; Fig. 7b ). A similar phenotype was observed in all four PI3KC2α-deficient mouse lines. 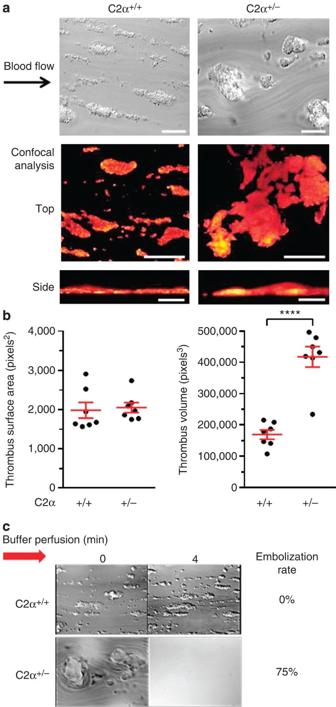Figure 7: PI3KC2α-deficient platelets develop large unstable thrombi. (a) Anticoagulated whole blood from littermate WT (C2α+/+) orPik3c2a+/gt1(C2α+/−) mice was perfused through microcapillary slides coated with type I collagen (250 μg ml−1) at a shear rate of 1,800 s−1for 3 min. Top panel: representative video stills of experiments showing thrombi forming in whole blood. Bottom panels: representative Z-series stacks of DiOC6-labelled thrombi (red) formed after 3 min and imaged via confocal microscopy, showing the larger overall size (top view) and increased height (side view) of C2α+/−thrombi. Scale bars, 100 μm. (b) Quantification of confocal-based thrombus reconstructions, showing thrombus surface area (pixels2; measured as adhesion area) and total thrombus volume (pixels3). Each data point is the average of eight fields of view from one microslide per mouse. Red bars are mean±s.e.m. ****P<0.0001 (unpaired, two-tailed, Student’st-test). (c) Representative images of thrombi from C2α+/+or C2α+/−mice after 3 min whole-blood flow over collagen at 1,800 s−1followed by perfusion of Tyrode’s buffer for the indicated times. Embolization of C2α+/+thrombi was never observed (0/31; experiments were stopped after 10 min buffer perfusion), yet 75% (6/8) of C2α+/−thrombi embolized within 4 min of buffer perfusion. Note the lack of cellular material remaining on the collagen substrate following thrombus embolization. Images are representative ofn≥8 experiments. Figure 7: PI3KC2α-deficient platelets develop large unstable thrombi. ( a ) Anticoagulated whole blood from littermate WT (C2α +/+ ) or Pik3c2a +/gt1 (C2α +/− ) mice was perfused through microcapillary slides coated with type I collagen (250 μg ml −1 ) at a shear rate of 1,800 s −1 for 3 min. Top panel: representative video stills of experiments showing thrombi forming in whole blood. Bottom panels: representative Z-series stacks of DiOC6-labelled thrombi (red) formed after 3 min and imaged via confocal microscopy, showing the larger overall size (top view) and increased height (side view) of C2α +/− thrombi. Scale bars, 100 μm. ( b ) Quantification of confocal-based thrombus reconstructions, showing thrombus surface area (pixels 2 ; measured as adhesion area) and total thrombus volume (pixels 3 ). Each data point is the average of eight fields of view from one microslide per mouse. Red bars are mean±s.e.m. **** P <0.0001 (unpaired, two-tailed, Student’s t -test). ( c ) Representative images of thrombi from C2α +/+ or C2α +/− mice after 3 min whole-blood flow over collagen at 1,800 s −1 followed by perfusion of Tyrode’s buffer for the indicated times. Embolization of C2α +/+ thrombi was never observed (0/31; experiments were stopped after 10 min buffer perfusion), yet 75% (6/8) of C2α +/− thrombi embolized within 4 min of buffer perfusion. Note the lack of cellular material remaining on the collagen substrate following thrombus embolization. Images are representative of n ≥8 experiments. Full size image Despite the increased thrombus growth, the most striking difference in thrombus dynamics was the propensity of thrombi from Pik3c2a +/gt1 mice to embolize from the collagen surface ( Fig. 7c ). Quantitative analysis revealed that 75% of the thrombi from Pik3c2a +/gt1 mice embolized within 4 min of blood perfusion, whereas none of the thrombi from Pik3c2a +/+ mice embolized. Thromboembolism appeared to be due to an inability of thrombi to maintain stable interaction with the collagen substrate rather than unstable platelet aggregation, as no disaggregation of the thrombus mass was observed and there were no intact platelets or residual platelet fragments on the collagen surface after embolization ( Fig. 7c ). Again, a similar phenotype was observed in all four PI3KC2α-deficient mouse lines. These findings indicate that PI3KC2α deficiency results in dysregulated platelet thrombus growth and stability. PI3KC2α deficiency enhances shear-dependent platelet adhesion Mobilization of internal membrane reserves is important for the increased platelet surface area that occurs during platelet shape change and spreading [32] . However, we found no evidence that the dilated OCS in PI3KC2α-deficient platelets represents additional membrane reserves in these cells. Specifically, no differences in filopodia formation or lamellipodia extension were observed between platelets from WT and Pik3c2a +/gt1 mice during adhesion to an immobilized fibrinogen matrix, and there were no differences in the surface area of these spread platelets ( Fig. 8a,b ). 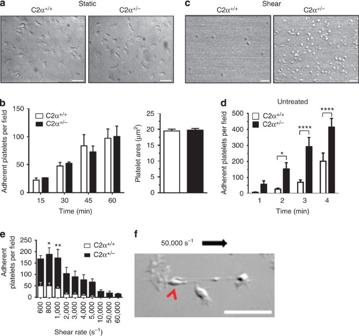Figure 8: Enhanced shear-dependent adhesion of PI3KC2α-deficient platelets. (a) Representative images (60 min) and (b) quantification of WT (C2α+/+) orPik3c2a+/gt1(C2α+/−) mice platelets adherent to a fibrinogen surface and their surface area at 60 min in the absence of blood flow (static). Bars are mean±s.e.m. fromn=3 independent experiments. No significant differences by genotype at any time point (unpaired, two-tailed, Student’st-test). (c) Representative images (2 min) and (d) quantification of platelets from C2α+/+or C2α+/−mice adherent to fibrinogen following perfusion of anticoagulated whole blood for 4 min at a rate of 600 s−1. Bars are mean±s.e.m. fromn=12–17 independent experiments. *P<0.05; ****P<0.0001 (unpaired, two-tailed, Student’st-test). (e) Whole blood from C2α+/+or C2α+/−mice was perfused over a fibrinogen surface for 3 min at 600 s−1, after which time the shear rate was incrementally increased every 1 min to the rates indicated sequentially on the abscissa, and the number of adherent platelets was quantified. Note the increased resistance to shear force of C2α+/−platelets: all C2α+/+platelets detached by 5,000 s−1, while some C2α+/−platelets withstood shear forces of up to 60,000 s−1. Data are mean±s.e.m. ofn=4–5. *P<0.05; **P<0.01 (two-way analysis of variance, with Bonferroni correction for multiple comparisons). (f) Representative image of a C2α+/−platelet adherent during exposure to a shear rate of 50,000 s−1(direction of flow indicated by black arrow) depicting elongated membrane tethers downstream of the cell body (red arrowhead). Scale bars, 5 μm. Figure 8: Enhanced shear-dependent adhesion of PI3KC2α-deficient platelets. ( a ) Representative images (60 min) and ( b ) quantification of WT (C2α +/+ ) or Pik3c2a +/gt1 (C2α +/− ) mice platelets adherent to a fibrinogen surface and their surface area at 60 min in the absence of blood flow (static). Bars are mean±s.e.m. from n =3 independent experiments. No significant differences by genotype at any time point (unpaired, two-tailed, Student’s t -test). ( c ) Representative images (2 min) and ( d ) quantification of platelets from C2α +/+ or C2α +/− mice adherent to fibrinogen following perfusion of anticoagulated whole blood for 4 min at a rate of 600 s −1 . Bars are mean±s.e.m. from n =12–17 independent experiments. * P <0.05; **** P <0.0001 (unpaired, two-tailed, Student’s t -test). ( e ) Whole blood from C2α +/+ or C2α +/− mice was perfused over a fibrinogen surface for 3 min at 600 s −1 , after which time the shear rate was incrementally increased every 1 min to the rates indicated sequentially on the abscissa, and the number of adherent platelets was quantified. Note the increased resistance to shear force of C2α +/− platelets: all C2α +/+ platelets detached by 5,000 s −1 , while some C2α +/− platelets withstood shear forces of up to 60,000 s −1 . Data are mean±s.e.m. of n =4–5. * P <0.05; ** P <0.01 (two-way analysis of variance, with Bonferroni correction for multiple comparisons). ( f ) Representative image of a C2α +/− platelet adherent during exposure to a shear rate of 50,000 s −1 (direction of flow indicated by black arrow) depicting elongated membrane tethers downstream of the cell body (red arrowhead). Scale bars, 5 μm. Full size image Membrane reserves also buffer surface tension following platelet exposure to haemodynamic shear stress [25] . We obtained two lines of evidence indicating that PI3KC2α-deficient platelets had dysregulated platelet adhesion under shear. First, Pik3c2a +/gt1 platelets adhered more efficiently to an immobilized fibrinogen matrix under physiologically relevant flow conditions ( Fig. 8c,d ). This enhanced adhesion was shear specific as Pik3c2a +/gt1 platelets adhered normally to fibrinogen in the absence of blood flow ( Fig. 8a,b ) and was observed in all four PI3KC2α-deficient mouse lines. Second, Pik3c2a +/gt1 platelets were more resistant to the detaching effects of sudden increases in shear, with significant cell adhesion maintained at shear rates as high as 50,000 s −1 ( Fig. 8e ). At these high shear rates, Pik3c2a +/gt1 platelets displayed considerable membrane deformity, with the development of elongated, thickened membrane protrusions ( Fig. 8f ). These studies define a role for PI3KC2α in regulating platelet adhesive function under conditions of haemodynamic shear stress. PI3KC2α links platelet internal membrane and tether formation The impact of haemodynamic shear stress on the structure of internal platelet membranes has not previously been examined. To investigate this, we exposed WT and PI3KC2α-deficient platelets to high shear stress using a cone-and-platelet viscometer. Ultrastructural analysis of platelets using transmission electron microscopy revealed a significant increase in the diameter of the OCS in both WT and PI3KC2α-deficient platelets following exposure to high shear ( Fig. 9a,b ). This shear-induced change in OCS structure correlated with the extent of shear-dependent platelet adhesion and occurred independent of platelet activation. Similarly, blocking the platelet activating effects of endogenously released ADP had only a minor effect on shear-dependent adhesion of Pik3c2a +/gt1 platelets to immobilized fibrinogen relative to littermate controls ( Fig. 9c ), suggesting that activation-independent events play an important role in regulating the shear-dependent adhesive function of PI3KC2α-deficient platelets. 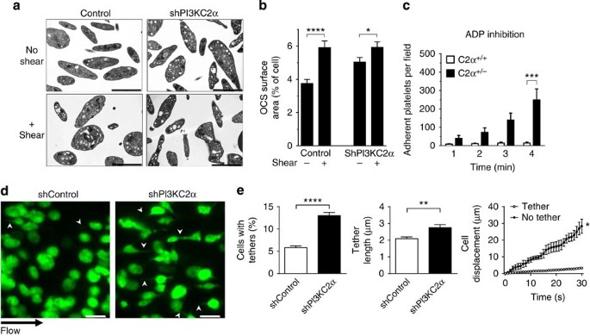Figure 9: PI3KC2α links platelet internal membrane to tether formation. (a) Representative TEM images (n=3) of activation-inhibited (theophylline, 10 mM) platelets from shPI3KC2α and shControl mice exposed to shear forces (+ shear) in a cone and plate viscometer (10,000 s−1, 5 min). Note dilated OCS in platelets from both genotypes exposed to shear. (b) Quantification of OCS surface area. Data are percentage total cell area and are mean±s.e.m. ofn=183–311 cells fromn=3 mice. *P<0.05; ****P<0.0001 (unpaired, two-tailed, Student’st-test). (c) Quantification of adherent platelets from C2α+/+or C2α+/−mice following perfusion of anticoagulated whole blood over a fibrinogen surface for 4 min at a rate of 600 s−1in the presence of apyrase, 2-methylthiolADP, and MRS2179 (ADP inhibition). Bars are mean±s.e.m. fromn=12 independent experiments. ***P<0.001 (unpaired, two-tailed, Student’st-test). (d) Representative images and (e) quantification of platelet tether formation. Anticoagulated whole blood from shPI3KC2α and shControl mice was perfused over a vWF surface for 3 min at a rate of 1,800 s−1. Note the formation of membrane tethers in platelets from shPI3KC2α mice. Data are mean±s.e.m. fromn=3 independent experiments. **P<0.01; ****P<0.0001 (unpaired, two-tailed, Student’st-test). Scale bars, 2 μm (a) and 5 μm (d). Figure 9: PI3KC2α links platelet internal membrane to tether formation. ( a ) Representative TEM images ( n =3) of activation-inhibited (theophylline, 10 mM) platelets from shPI3KC2α and shControl mice exposed to shear forces (+ shear) in a cone and plate viscometer (10,000 s −1 , 5 min). Note dilated OCS in platelets from both genotypes exposed to shear. ( b ) Quantification of OCS surface area. Data are percentage total cell area and are mean±s.e.m. of n =183–311 cells from n =3 mice. * P <0.05; **** P <0.0001 (unpaired, two-tailed, Student’s t -test). ( c ) Quantification of adherent platelets from C2α +/+ or C2α +/− mice following perfusion of anticoagulated whole blood over a fibrinogen surface for 4 min at a rate of 600 s −1 in the presence of apyrase, 2-methylthiolADP, and MRS2179 (ADP inhibition). Bars are mean±s.e.m. from n =12 independent experiments. *** P <0.001 (unpaired, two-tailed, Student’s t -test). ( d ) Representative images and ( e ) quantification of platelet tether formation. Anticoagulated whole blood from shPI3KC2α and shControl mice was perfused over a vWF surface for 3 min at a rate of 1,800 s −1 . Note the formation of membrane tethers in platelets from shPI3KC2α mice. Data are mean±s.e.m. from n =3 independent experiments. ** P <0.01; **** P <0.0001 (unpaired, two-tailed, Student’s t -test). Scale bars, 2 μm ( a ) and 5 μm ( d ). Full size image The pulling of membrane tethers from the surface of platelets by hemodynamic shear stress is an important activation-independent event regulating platelet adhesion [35] . Notably, the kinetics of membrane tether formation are regulated in part by membrane reserves [25] . Consistent with this, platelets from shPI3KC2α mice pulled twice as many tethers under shear relative to shControl mice ( Fig. 9d,e ). These tethers were longer and supported more sustained platelet adhesion relative to platelets without tethers ( Fig. 9d,e ). Taken together, these findings suggest that shear-dependent structural changes in the platelet internal membranes enhance membrane tether formation and adhesion under flow in PI3KC2α-deficient platelets. This study provides the first detailed analysis of the role of the class II PI3Ks in regulating platelet function. While we have shown that PI3KC2β is the major class II PI3K isoform expressed in platelets, no significant function of this enzyme was detected in these cells. In contrast, we demonstrated using four distinct mouse genetic models of PI3KC2α deficiency that PI3KC2α has a role in regulating platelet function that is sufficient to impact on in vivo arterial thrombosis. Despite this significant in vivo platelet function defect, we could find no evidence that PI3KC2α has an important signalling role in platelets. Rather, our studies indicate that PI3KC2α regulates the structure of the internal membrane reserves of platelets (OCS). The major effect of this membrane structural defect relates to shear-dependent changes in platelet adhesive function that result in the formation of large, unstable, platelet thrombi in a range of ex vivo and in vivo thrombosis models. Overall, these studies are the first to demonstrate a role for PI3Ks in regulating the internal membrane reserves of cells, and suggest a potentially important role for the OCS in controlling the adhesive function of platelets. While our studies confirmed the expression of both PI3KC2α and PI3KC2β in platelets, we did not identify an acute signalling role for either enzyme in these cells. Specifically, the levels of 3-PPIs in PI3KC2α- or PI3KC2β-deficient platelets were unaltered in resting and agonist-stimulated platelets, and all soluble agonist-induced platelet functional responses examined were normal. While spatial changes in PI(3)P accumulation can be difficult to detect when performing phospholipid analysis on whole-cell lysates, the lack of a direct signalling function of class II PI3Ks is supported by our observations that neither PI3KC2α nor PI3KC2β contributed to a broad range of agonist-induced, signalling-dependent, platelet activation events, including shape change, integrin α IIb β 3 activation, aggregation or the release of secretory granules. One previous report has suggested that PI3KC2β promotes PI(3,4)P 2 accumulation in human platelets following activation and integrin α IIb β 3 ligation [30] . However, we could find no evidence for an important role for PI3KC2β in regulating PI(3,4)P 2 levels or integrin α IIb β 3 outside-in signalling events linked to sustained platelet aggregation or cytoskeletal changes necessary for platelet spreading. Furthermore, the demonstration of normal haemostasis in Pik3c2 β −/− mice, even with anticoagulation, as well as a normal thrombotic response, does not support an important role for PI3KC2β in regulating the in vivo function of platelets. In contrast, our studies on a series of PI3KC2α-deficient mice demonstrated marked changes in platelet adhesive function in the setting of ex vivo and in vivo thrombosis. We observed a shear-dependent increase in platelet adhesion that caused dysregulated thrombus growth and compromised overall thrombus stability. There were several striking features of this phenotype. First, partial reduction in PI3KC2α expression was sufficient to dysregulate platelet function, with this phenotype observed in two Pik3c2a heterozygous mouse lines and a Pik3c2a hypomorph. Such a ‘gene–dosage effect’ perturbing primary haemostasis and arterial thrombosis is infrequently observed in platelet-dependent phenotypes, but presumably reflects the altered membrane structures apparent in all PI3KC2α-deficient mouse lines. Second, the increased adhesion was primarily manifested under shear conditions, with no changes in platelet adhesion observed in the absence of the shear forces provided by flowing blood. Third, PI3KC2α-deficient platelets efficiently formed stable adhesion contacts with immobilized fibrinogen without the requirement for platelet co-stimulation by soluble agonists, most notably ADP. This effect was striking considering that signals generated by the fibrinogen–integrin α IIb β 3 interaction are relatively weak [36] , [37] , with full platelet activation requiring the release of dense granule ADP [36] , [37] . We could find no evidence for a change in integrin α IIb β 3 affinity in resting or agonist-stimulated PI3KC2α-deficient platelets that would explain the ability of these platelets to maintain sustained adhesive interactions with the fibrinogen substrate over a broad shear range. Rather, it was notable that structural alterations in the platelet internal membrane reserves, the OCS, could be induced in a similarly shear-dependent, activation-independent manner. This observation, along with the demonstration that activation-independent membrane tether formation was dysregulated in PI3KC2α-deficient platelets, suggests a potentially important role for membrane structural changes in regulating the adhesive function of platelets under conditions of haemodynamic shear stress. Membrane reserves are important components of a variety of haematopoietic cells [23] , providing a readily available source of lipid bilayer for the rapid expansion of plasma membrane. In addition to their structural function, membrane reserves also play an important role in buffering major fluctuations in plasma membrane tension [25] , since plasma membranes have limited capacity to stretch before undergoing lysis [38] . It is known that the tension associated with platelet spreading leads to collapse of the OCS and total evagination of the membrane reserve [39] . Thus, it is conceivable that shear effects on the platelet plasma membrane may lead to alterations in the platelet OCS that modify platelet adhesive function. Although it remains to be established whether changes in membrane tension, deregulation of membrane trafficking from the OCS to the cell surface and/or alterations in membrane tether formation underlie the increased adhesive function of PI3KC2α-deficient platelets, it is worth noting that integrin α IIb β 3 receptors are highly expressed in the membrane of the OCS [39] . Furthermore, a growing body of evidence has accumulated from the study of shear-dependent adhesion of other haematopoietic cells, particularly neutrophils [40] , [41] , that dynamic changes in the plasma membrane, some of which involves membrane reserves, have a profound impact on cell adhesion. The studies presented here suggest for the first time that PI3KC2α plays an important role in regulating the structure of internal membranes that occur independently of changes in the overall amount of membrane reserve. PI3KC2α is preferentially localized to endosomes and the trans -Golgi network with evidence for an important role for both PI(3)P and PI(3,4)P 2 in regulating membrane dynamics [16] , [42] , [43] . Given the poor expression levels of PI3KC2α in platelets, the lack of signalling from PI3KC2α detected in platelets and the structural defect in the internal membranes of PI3KC2α-deficient megakaryocytes, it is possible that the effects of 3-PPI on OCS structure in the platelet occur secondary to membrane changes in the developing megakaryocyte. On this point, two recent studies have demonstrated that the phosphoinositide, PI(4,5)P 2 , plays an important role in regulating the development and structure of the internal membrane of the megakaryocyte, the DMS, and in maintaining the integrity of the membrane–cytoskeleton link of platelets [44] , [45] . Although the platelet phenotype observed in our studies is clearly distinct from that of these previous studies, based on findings related to clathrin-mediated endocytosis where the conventional phosphoinositide, PI(4,5)P 2 , acts in concert with 3-PPIs to regulate endosome development and maturation [42] , [46] , it is possible that a similar co-operative function operates between PI(4,5)P 2 and 3-PPIs to regulate internal membrane reserves in platelets and megakaryocytes. To our knowledge, the novel mouse models of PI3KC2α deficiency generated here provide the first example of a specific, isolated, defect in OCS structure. Despite several existing examples in which platelets display a dilated [47] , [48] or otherwise disrupted [49] , [50] OCS, additional alterations in platelet ultrastructure are present in each instance. Clinical conditions in which the OCS structure is disrupted have not been explicitly determined, although a dilated OCS has been reported in patients with the prothrombotic Budd–Chiari syndrome [48] as well as the macrothrombocytic May–Hegglin anomaly [51] . Again, the changes in OCS in the platelets of these patients are accompanied by other ultrastructural variations that may contribute to the platelet functional defects observed in these clinical conditions. Whether or not a selective disruption of the OCS is sufficient to cause symptomatic bleeding in humans is unknown, although it is worth noting that the impact on in vivo haemostatic function in mice with a partial deficiency of PI3KC2α ( Pik3c2a +/gt1 ) was similar to that observed in WT mice treated with aspirin, and that near-complete deficiency of PI3KC2α (shPI3KC2α) resulted in a more severe defect in primary haemostatic function. Finally, our study provides further evidence for divergent roles of the class II PI3K isoforms. PI3KC2α, PI3KC2β and PI3KC2γ have different expression patterns, respond to different extracellular stimuli and appear to have distinct downstream cellular signalling functions [1] , [10] , [11] , [12] , [13] , [52] , [53] . We have used a novel genetic approach to reveal a specific function for PI3KC2α in regulating the structure of the internal membrane reserves of platelets. Unexpectedly, these structural changes are associated with marked alterations in platelet adhesive behaviour sufficient to impact on the primary haemostatic and prothrombotic function of these cells. These studies provide new insights into the role of internal membrane reserves in regulating the shear-dependent adhesive function of platelets necessary for stable arterial thrombus formation. Mice All mice used in this study were backcrossed ≥5 generations onto a C57Bl/6 genetic background (that is, ≥98%) and maintained on a 12-h light/dark cycle with food and water ad libitum. All studies were littermate controlled and were performed using mice of either gender between the ages of 6 and 20 weeks. All studies were approved by the Alfred Medical Research and Education Precinct Animal Ethics Committee (approvals E/0475/2006/M, E/0693/2008M and E/0937/2009/M). Pik3c2b −/− mice [9] and hypomorphic PI3KC2α mice [10] have been generated previously. Generation of Pik3c2a −/− mice Disruption of murine Pik3c2a (GenBank accession number NM_011083) and subsequent generation of Pik3c2a −/− mice was achieved using a conventional gene trapping approach [54] . The distinct 129Ola embryonic stem cell clones CJ0058 and AS0568 from the International Gene Trap Consortium [55] were used, in which disruption of Pik3c2a was achieved using a gene trap construct consisting of a splice acceptor, followed by a β-galactosidase reporter and 3′ polyadenylation stop signal. The insertion site of the gene trap vector in each clone was determined by 5′ RACE and confirmed by reverse transcription (RT)–PCR: insertion of the gene trap was into intron 19 for clone CJ0058 ( Pik3c2a gt1 ) and intron 25 for clone AS0568 ( Pik3c2a gt2 ; Fig. 2a ). A clonal embryonic stem cell population was confirmed by X-gal staining of cultured cells before microinjection into C57Bl/6 blastocysts to generate chimaeric mice. Male chimaeras were bred to female C57Bl/6 mice to confirm germline transmission of the mutation and to generate heterozygous mice. Genotyping of Pik3c2a alleles was performed by RT–PCR ( Fig. 2b ), using the following primer sequences: common forward (5′-AAGTAAGGCAGGCTAGTGGA-3′), WT reverse (5′-GTCAGAGGTAAGCACAAAAGG-3′) and mutant reverse (5′-AGTATCGGCCTCAGGAAGATCG-3′). Generation of shPI3KC2α mice The generation of bitransgenic mice allowing inducible and reversible shRNA-based knockdown of PI3KC2α was performed using published techniques [56] , [57] . Ten mir30-based shRNAs were screened for their ability to reduce PI3KC2α protein expression after retroviral transduction of mouse fibroblasts, and the most effective shRNA was cloned into a tet-responsive element-GFP-shRNA (TRE-GFP-shRNA) vector [58] that was targeted to the type I collagen (Colla1) locus in KH2 embryonic stem cells using an FLP-mediated recombination strategy [59] . Hygromycin-resistant clones were isolated, and successfully targeted cells were determined by doxycycline-induced GFP expression and were injected into C57BL/6 mouse blastocysts. Resultant male chimaeras were crossed to female C57BL/6 mice. Confirmed TRE-GFP-shRNA mice were then crossed with CMV-rtTA mice to generate bitransgenic mice, which were maintained through C57BL/6 backcrossing. The TRE-GFP-shRNA transgene was detected via PCR using the forward primer: (5′-TAACTTCTTCACTGCTTCTGTTGC-3′) and a common reverse primer: (5′-GAAAGAACAATCAAGGGTCC-3′) yielding a 210-bp product. The CMV-rtTA transgene was detected via PCR using forward primer (5′-GCTTGGTGTAGAGCAGCCTACAC-3′) and reverse primer (5′-CAGCGCTGAGTGCATATAACGCG-3′), yielding a 311-bp product. Mice were administered doxycycline in their food (600 mg kg −1 ; Specialty Feeds). Analysis of mouse embryos Pregnancies from heterozygous intercrosses were timed by the presence of vaginal plugs and the embryos from pregnant females harvested at 7.5–13.5 days post coitum (dpc) under a dissecting microscope. Whole-mount pictures were taken with an Olympus IX81 or Zeiss AxioCam HRc. To confirm loss of protein expression, western blot analysis was performed as described below on whole-cell lysates prepared from 8.5 dpc embryos and probed using an anti-PI3KC2α antibody (1:250, BD Biosciences, San Diego, CA), anti-PI3KC2β antibody (1:1,000, BD Biosciences) or anti-β-actin antibody (1:1,000, Abcam). Mouse platelet isolation Platelets were isolated from blood that was drawn into hirudin (800 U), treated with acid-citrate-dextrose and a platelet wash buffer (4.3 mM K 2 HPO 4 , 4.3 mM NaHPO 4 , 24.3 mM NaH 2 PO 4 , 113 mM NaCl, 5.5 mM D-glucose and 10 mM theophylline; pH 6.5; containing 0.05% BSA, 800 U total hirudin and 0.02 U ml −1 apyrase), and platelets isolated via centrifugation and resuspended at the required concentration in Tyrode’s buffer containing BSA (5 mg ml −1 ), Ca 2+ (1 mM) and apyrase (0.02 U ml −1 ; refs 33 , 34 ). Western blotting Reduced and denatured protein samples were separated via SDS–PAGE (7.5%) and transferred to PVDF membranes for probing with antibodies against PI3KC2α (1:250), PI3KC2β (1:1,000), PI3KC2γ (1:100) or β-actin (1:1,000; all obtained from BD Biosciences). Scans of uncropped blots are shown in Supplementary Fig 8 . 3-PPI generation Isolated platelets were resuspended in phosphate-free Tyrode’s buffer containing the platelet activation inhibitor theophylline (10 mM) and labelled with 0.3 mCi ml −1 inorganic [ 32 P]H 3 PO 4 for 2 h at 37 °C. Unincorporated [ 32 P]H 3 PO 4 was removed before 32 P-labelled platelets were stimulated with either thrombin (1 U ml −1 ), CRP (10 μg ml −1 ) or vehicle for nominated time points and then lysed and lipids extracted and separated by high-performance liquid chromatography [60] . Phosphoinositide peaks co-eluting with PtdIns(3)P, PtdIns(3,4)P 2 and PtdIns(3,4,5)P 3 standards were integrated and expressed as a percentage of total phospholipid applied. Surface expression of platelet-specific glycoproteins Whole blood was stained with fluorescein isothiocyanate-conjugated antibodies against the platelet-specific glycoproteins, GPIbα (clone Xia.G5), GPIbβ (Xia.C3), GPIIbIIIa (Leo.F2) or GPVI (JAQ1) and analysed via fluorescence-activated cell sorting. All antibodies were from EMFRET and all were used at a 1 in 5 dilution in blood diluted 1 in 20 with Tyrode’s buffer. Platelet aggregation Aggregation of isolated platelets (2 × 10 8 ml −1 ) was determined via light transmission (AggRAM, Helena Laboratories) in the presence of fibrinogen (500 μg ml −1 ) and in response to CRP (1 and 5 μg ml −1 ), ADP (0.5 and 5 μM) and a PAR4-activating peptide (AYPGKF; 50 and 100 μM). Integrin α IIb β 3 activation A mixture of isolated platelets (5 × 10 7 ml −1 ) and Oregon-green fibrinogen (20 μg ml −1 ) were stimulated (10 μg ml −1 CRP or 100 μM PAR4-activating peptide) and the response terminated at nominated time points by the addition of 2% paraformaldehyde (PFA). Oregon-green fibrinogen binding was analysed via FACS. Alpha and dense granule release For alpha granule release, P-selectin expression on the platelet surface was analysed as described above (fibrinogen-binding assay), using a directly conjugated anti-P-selectin antibody (1 μg ml −1 ; BD Biosciences). For dense granule release, isolated platelets were loaded with 14 C-labelled serotonin (0.017 MBq), washed and release of 14 C-serotonin measured in response to agonist stimulation using a scintillation counter (Beckman LS 6000). In vivo haemostasis assays Tail transection bleed times were performed as described [61] . Briefly, mice were anaesthetized with tribromoethanol (Avertin, Sigma, 250 mg kg −1 intraperitoneal) and their tails were transected 5 mm from the tip with a scalpel blade. The bleeding end was immediately immersed in saline at 37 °C and time to cessation of flow (stoppage for >2 min) was measured. Template tail bleed times were performed on mice anaesthetized with sodium pentobarbitone (Nembutal, Boehringer Ingelheim; 40 mg kg −1 intraperitoneal), maintained at 37 °C via a heat pad and ventilated using tracheal intubation. In some experiments, hirudin (Refludan, Celgene), aspirin (Solprin, Reckitt Benckiser) or their vehicle (volume matched 0.9% saline) were administered via the jugular vein 5 min before tail incision. A scalpel blade was used to generate a lateral incision 5 mm long and 2 mm deep, 1 cm from the tip of the mouse’s tail. Bleeding was assessed by blotting tissue against the wound site every 30 s for 15 min or until no further blood was detected on the tissue for two consecutive blotting periods. In vivo thrombosis model The electrolytic model of thrombosis was performed essentially as described [33] , [62] , [63] . Mice were anaesthetized using sodium pentobarbitone and a flow probe (0.5 mm inner diameter) linked to a flow meter (TS420, Transonic Systems) placed around the exposed left carotid artery to record blood flow using PowerLab Chart (v. 5.0, AD Instruments). A constant current lesion maker (Model D.C.LM5A, Grass Instruments) was used to deliver 18 mA for 2 min to the carotid artery via a platinum electrode—the minimal current required to reliably produce a stable occlusive thrombotic event in untreated, WT mice. Bone marrow transplantation Six- to 10-week-old WT and Pik3c2a +/gt1 mice were used as both donors and recipients in bone marrow transplant experiments. Recipients were exposed to whole-body irradiation with two doses of 550 rad, 3 h apart and were reconstituted with 1 × 10 6 donor bone marrow cells intravenous (i.v.). To assess the extent of haematopoietic reconstitution, the relative expression of the CD45 isotypes on circulating leukocytes were examined using directly conjugated antibodies against CD45.1 and CD45.2 (Abcam). Transmission electron microscopy Platelet and megakaryocyte ultrastructure was analysed via transmission electron microscopy (TEM), essentially as described [64] . Briefly, isolated platelets were fixed in 2% glutaraldehyde, 2.5% PFA, post fixed in 2% osmium tetroxide and dehydrated through a graded ethanol series before being embedded in Spurrs resin. In situ bone marrow megakaryocytes were prepared by perfusion–fixation of anaesthetized mice with 2% glutaraldehyde, 2.5% PFA via the ascending aorta at a rate of 20.4 ml h −1 (Perfusor Compact S, Braun). The femurs were excised and immersion fixed for a further 4 h, rinsed in PBS and decalcified in 10% EDTA for 7 days at 4 °C before post fixation, dehydration and embedding as above. Ultrathin sections of all samples were cut with a diamond knife (Diatome) on an ultramicrotome (Leica) and stained with methanolic uranyl acetate and lead citrate before TEM (JEOL 1011). Images were recorded with a MegaView III CCD (Soft Imaging Systems). For ruthenium red staining, isolated platelets were fixed in 2.5% glutaraldehyde with 1 mg ml −1 ruthenium red in 0.1 M cacodylate buffer, rinsed in 0.1 M cacodylate buffer, and then post fixed with 1% osmium tetroxide with 1 mg ml −1 ruthenium red before sectioning. In some experiments, isolated platelets (3 × 10 8 ml −1 in platelet wash buffer (pH 6.5) containing theophylline (10 mM), hirudin (800 U) and apyrase (0.02 U ml −1 )) were sheared at 10,000 s −1 for 10 min in a cone-and-plate viscometer before TEM analysis as above. Megakaryocyte ploidy analysis Whole bone marrow suspensions isolated from shPI3KC2α and shControl mice were prepared in PBS containing sodium citrate (0.38%) and BSA (0.5%) and 1 × 10 7 cells labelled for 15 min at room temperature with 1.5 μg DyLight-650-conjugated monoclonal antibody against CD42b (rat anti-mouse glycoprotein Ibα; EMFRET), washed twice in PBS-citrate-BSA buffer and fixed with ethanol (70% v/v in PBS) for 1 h at 4 °C. The cells were then stained in 500 μl propidium iodide/RNase staining buffer (BD Pharmingen) for 15 min at room temperature. The ploidy distribution of CD42b+ population was determined by two-colour flow cytometry (LSRII, Beckton Dickinson) and analysis (FlowJo). Proplatelet production Whole bone marrow flushed from the femura and tibiae of 6- to 8-week-old shPI3KC2α and littermate control mice was plated in complete DMEM (containing 10% fetal calf serum, 2 mM L-glutamine and 50 U ml −1 penicillin/streptomycin) in the presence of thrombopoietin and cultured at 37 °C in 5% CO 2 for 5 days, after which the percentage of proplatelet-producing megakaryocytes was determined by light microscopy. In vivo platelet half-life Biotinylation of the surface of circulating platelets was performed by i.v. injection of N -hydroxysuccinimidobiotin (30 μg g −1 EZ-Link NHS-biotin; Thermo Scientific). Submandibular bleeds were performed into K2-EDTA tubes at various time points after injection and isolated platelets were stained with Phycoerythrin (PE)-labelled streptavidin (0.2 μg ml −1 ; Jomar Biosciences) for 30 min at 37 °C and the percentage of biotinylated platelets determined by flow cytometry (FACSCalibur; Beckton Dickinson). In vivo platelet production Immune-mediated platelet depletion was performed on shPI3KC2α and littermate control mice by i.v. injection of rabbit anti-mouse thrombocyte serum (0.2 μl g −1 ; Cedarlane). Submandibular bleeds were performed into K2-EDTA tubes at various time points after injection and whole-blood platelet counts were performed (Hemavet 950 S, Drew Scientific). Ex vivo thrombosis and platelet adhesion assays Glass microslides (0.1 × 1.0 mm, VitroCom) were washed in nitric acid, rinsed with dH 2 O and sonicated for 15 min before coating with either bovine type I collagen (250 μg ml −1 diluted in 10 mM acetic acid for ≥2 h) or fibrinogen (100 μg ml −1 , overnight). For thrombus formation on collagen, mouse whole blood collected in hirudin (800 U) was perfused through coated slides at 37 °C for 3 min at 1,800 s −1 and thrombus formation and platelet adhesion monitored via an inverted Leica DMIRB microscope using a × 63 water objective and recorded in real-time using a DAGE-MTI CCD camera (300 ETRCX). For analysis of thrombus surface area and volume, platelets deposited on microslides were stained with DiOC 6 (1 μM) and sectioned using confocal microscopy (Leica TCS NT). Surface area was defined as the area of the thrombus base covering the collagen surface, as measured on the first confocal section (1 μm) and expressed as pixels 2 (ImageJ). Thrombus volume was defined as the sum of the surface areas of the Z-series stack and was expressed as pixels 3 . For platelet interaction with fibrinogen, mouse whole blood collected in hirudin (800 U) was perfused for 3 min at 600 s −1 . Platelet adhesion was determined by counting the number of platelets attached to the matrix for ≥10 s at a given time point. Platelets were defined as stationary if they moved <1 cell diameter in 10 s. In some experiments, perfusion of blood was followed by perfusion of Tyrode’s buffer at incremental increases in shear rate 1 min apart and tethered platelets were monitored until detachment. In further experiments, blood was incubated with a combination of the ADPase apyrase (0.02 U ml −1 ), the P2Y1 antagonist MRS2179 (100 μM) and the P2Y12 antagonist 2-methylthio-AMP (10 μM) for 10 min before perfusion over fibrinogen for 3 min at 600 s −1 and platelet adhesion quantified as above. Static adhesion of platelets to immobilized fibrinogen was performed on glass coverslips coated with fibrinogen (10 μg ml −1 ) for ≥3 h at 4 °C. Non-immobilized fibrinogen was removed with Tyrode’s and exposed glass was blocked with 2% BSA. Washed platelets resuspended in Tyrode’s buffer at 5 × 10 7 ml −1 were placed on the coverslips and allowed to spread for 15, 30, 45 or 60 min. Non-adherent platelets were then removed with a Tyrode’s buffer wash and adherent platelets were fixed using 2% PFA for 30 min and imaged using an inverted Leica DMIRB microscope with a × 100 oil objective. Membrane tether formation by platelets was examined in hirudin-anticoagulated whole blood perfused over von Wiilebrand factor (vWF)-coated microchannels at 1,800 s −1 . Polydimethylsiloxane (PDMS) microchannels were coated with a capturing anti-vWF antibody (20 μg ml −1 ; Merck Millipore AB7356) for 1 h at room temperature, flushed with Tyrode’s buffer, blocked with BSA (2% w/v), coated with mouse platelet poor plasma for 2 h and then flushed with Tyrode’s buffer before use. Platelet tether formation was examined for 3 min with concurrent TIRF widefield imaging (Olympus IX83; × 150 oil immersion objective, numerical aperture 1.45; Photometrics Evolve Delta Camera; Cellsens 1.9 software). Videos were analysed offline using ImageJ software for the number of platelets forming membrane tethers and platelet rolling velocity. Statistical analyses All statistical analyses were carried out using Prism software (v 6, GraphPad). Statistical significance ( P <0.05) was determined by one of log rank, analysis of variance or t -test, as indicated in the figure and table legends. Sample sizes were determined to provide a Power of 0.8 using an α-error level of 0.05. How to cite this article: Mountford, J. K. et al. The class II PI 3-kinase, PI3KC2α, links platelet internal membrane structure to shear-dependent adhesive function. Nat. Commun. 6:6535 doi: 10.1038/ncomms7535 (2015).